Contemporary and historical separation of transequatorial migration between genetically distinct seabird populations Pelagic seabirds are highly mobile, reducing the likelihood of allopatric speciation where disruption of gene flow between populations is caused by physically insurmountable, extrinsic barriers. Spatial segregation during the non-breeding season appears to provide an intrinsic barrier to gene flow among seabird populations that otherwise occupy nearby or overlapping regions during breeding, but how this is achieved remains unclear. Here we show that the two genetically distinct populations of Cook's petrel ( Pterodroma cookii ) exhibit transequatorial separation of non-breeding ranges at contemporary (ca. 2–3 yrs) and historical (ca. 100 yrs) time scales. Segregation during the non-breeding season per se appears as an unlikely barrier to gene flow. Instead we provide evidence that habitat specialization during the non-breeding season is associated with breeding asynchrony which, in conjunction with philopatry, restricts gene flow. Habitat specialization during breeding and non-breeding likely promotes evolutionary divergence between these two populations via local adaptation. Divergent migratory behaviours to and from breeding sites have led to the disruption of gene flow among populations in many species [1] , [2] , contributing to reproductive isolation under the classic model of allopatric speciation [3] . In terrestrial environments, genetic differentiation among migratory populations is frequently paralleled by extrinsic (for example, mountain ranges) and intrinsic (for example, timing of dispersal, inherited migratory direction and host use by parasites) barriers that restrict gene flow and facilitate divergence via genetic drift and/or selection [4] , [5] , [6] . However, the nature of the extrinsic and intrinsic barriers that disrupt gene flow among populations of marine animals has only recently begun to be investigated [7] , [8] and remains poorly known for many highly mobile taxa [8] , [9] . Seabirds undertake the longest known migrations on Earth, routinely crossing hemispheres between breeding and non-breeding habitats within ocean basins [10] , [11] . As a result of this extreme mobility, seabirds experience few apparent physical barriers to dispersal. Thus, seabirds can potentially visit and ultimately breed on islands thousands of kilometres from their natal colony, which may contribute to a lack of genetic structure observed in several species [12] , [13] , [14] , [15] . Yet, other seabird species show surprisingly high levels of population genetic structure [8] , [16] , [17] , [18] and intrinsic barriers to gene flow appear to have an important role in the evolution of seabird diversity [4] , [18] , [19] , [20] , [21] , [22] . For example, given the strong tendency for seabirds to return to their natal site to breed, natal philopatry has been proposed as one such a barrier to gene flow [19] . However, given that not all seabirds exhibit strong genetic structure, it is unlikely to be the sole driver of population differences. A recent meta-analysis suggests that segregation of non-breeding distributions may be a key determinant of genetic structure among seabird populations [8] , but how occupying disjunct non-breeding distributions can restrict gene flow remains unclear. Although advances in tracking technology have improved our ability to record the long-distance movements of seabirds at sea [20] , few studies have examined the non-breeding segregation amongst seabird populations that occupy nearby or overlapping regions during the breeding season [11] , [21] . Accordingly, the role of seasonal movements in shaping the genetic structure of seabird populations, and the persistence of these movement patterns at the timescale of generations, remain unknown. Such information is vital for providing insights into behavioural and ecological mechanisms underlying the diversification of highly mobile taxa, including those within oceanic environments. Pterodroma cookii (Cook's petrel; Procellariiformes: Procellariidae (Gray, 1843)), are pelagic seabirds that breed exclusively on two islands at the northern and southern extremes of their historic range within the New Zealand archipelago [22] : Little Barrier Island (LBI) and Codfish Island (CDF), respectively [23] , [24] . When breeding, P. cookii range within the south-west Pacific and Tasman Sea, with overlapping foraging ranges centred around their respective breeding colonies [25] . Shipboard observations indicate that after breeding, P. cookii are trans-equatorial and trans-Pacific migrants, with sightings concentrated in the North Pacific (North-Pacific Convergence and centrally along Baja California: BC) and in the South Pacific (Humboldt Current: HC) Oceans [26] . On the basis of body size and plumage characteristics, in 1929, Murphy [27] distinguished between smaller P. cookii cookii that were collected in the North Pacific and assigned to the breeding population at LBI, and the larger P. cookii orientalis , of unknown breeding origin, collected south of the Equator, off the coast of Peru. Subsequently, Falla [28] observed that the plumage and morphological characteristics of P. c. orientalis were consistent with juveniles of P. c. cookii from the breeding population at CDF that was discovered in 1934 (ref. 24 ). In addition to differences in body size, body mass and the potential for non-breeding birds to occupy disjunct habitats [5] , [26] , [29] , birds on LBI and CDF exhibit a 1-month asynchrony in breeding phenology [5] and are genetically distinct [6] . These combined observations strongly suggest that gene flow between the two extant P. cookii populations is highly restricted. Thus, P. cookii is an ideal study species to explicitly examine whether and how occupying disjunct non-breeding distributions can restrict gene flow among seabird populations. Here we combined geolocator-based tracking with an isotopic (δ 13 C and δ 15 N) and genetic (mitochondrial cytochrome oxidase subunit 1) comparison of modern breeding birds, and historical specimens (that is, museum skins), to test the hypothesis of transequatorial separation of the two P. cookii breeding populations at varying temporal scales. Specifically, we tested the predictions that contemporary P. cookii populations, tracked over a complete annual cycle, would exhibit divergent non-breeding distributions, habitat use and foraging patterns; this divergence would be consistent between contemporary cycles (ca. 2–3 years) as revealed by stable isotope analyses; the stable isotope signatures of historical specimens of unknown breeding provenance, collected ca. 100 years ago from the two non-breeding oceanic regions used by contemporary populations, would match those of modern samples; and that genetic analysis would clearly assign origin of breeding population for these museum specimens and confirm divergence in transequatorial migration of the P. cookii populations over historical timescales. This combination of tracking, museum-based investigation, and elemental and molecular analyses presents a novel opportunity to evaluate how differences in contemporary and historical migratory behaviour can contribute to the diversification of a highly mobile marine species. Population movements Consistent with the prediction that contemporary tracked P. cookii would exhibit divergent non-breeding distributions, our analysis reveals that birds tracked between consecutive breeding seasons using light-based geolocation loggers (hereafter called loggers) between 2007 and 2009 from LBI ( n =11: female (♀)=5, male (♂)=6) and CDF ( n =11: ♀=6, ♂=5) exhibited transequatorial separation of their non-breeding habitats within the Pacific Ocean ( Fig. 1 , Supplementary Fig. S1 ). This contrasts with previous studies of other transequatorial migrants, including related Procellariiform seabirds, which showed substantial overlaps in space use and mixing during the non-breeding period of individuals that originated from different breeding populations [10] , [11] , [29] . Post-breeding LBI P. cookii (tracked for 389±49 s.d. days) completed an anti-clockwise migration of 48,037±7953 s.d. km within the North and South Pacific Ocean. Birds tracked from LBI moved east, then north across the equator to reach core non-breeding distributions within the California and North-Pacific currents (approximately 35°N) in 34±8 s.d. days. Pre-breeding migration returning to New Zealand waters was completed in 20±5 s.d. days ( Fig. 1 ) on a direct southwest route. In contrast, post-breeding CDF P. cookii (tracked for 450±3 s.d. days) migrated within the South Pacific Ocean (37,813±6,920 s.d. km) moving east and then north within the Humboldt Current to reach core non-breeding distributions off the Peruvian Coast (approximately 15°S) in 19±5 s.d. days. Pre-breeding migration returning to New Zealand was again completed in 20±5 s.d. days through a south-western corridor, north of the region traversed during post-breeding movements. Consistent with their breeding timetables, the migration schedule of both the P. cookii populations was asynchronous; LBI birds commenced post- and pre-breeding migrations approximately 1 month before CDF birds (post-breeding 11 March±12 s.d. days versus 8 April±15 s.d. days (t (18) =−4.67, P <0.0001); pre-breeding 5 Sept±10 s.d. days versus 20 Oct±6 s.d. days (t (15) =−11.85, P <0.0001)). 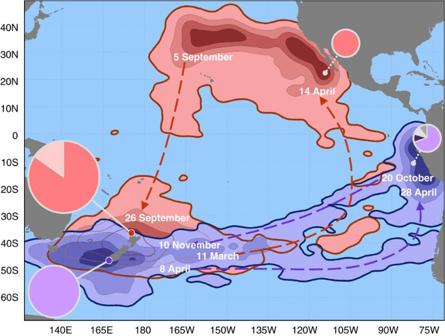Figure 1: Pacific migrations of trackedP. cookii. Movements ofP. cookiibreeding on LBI (red circle, North Island) and CDF (purple circle, South Island), New Zealand. Approximate post-breeding and pre-breeding migration routes of tracked LBI (red dashed lines) and CDF (purple dashed lines) birds begin and end with mean migration departure and arrival dates (white text). Red and purple tones, and associated contour lines, represent the 95, 75, 50 and 25% kernel estimates for LBI and CDF birds respectively. Pie charts show the geographic distribution of cytochromecoxidase subunit 1 mtDNA haplotypes sequenced from modernP. cookiipopulations (charts attached to LBI and CDF colony locations) and historicalP. cookiiskins collected in the North (BC) and South Pacific (HC) Ocean in 1905 and 1913 respectively (charts attached to white circles showing approximate collection location). Pie chart size reflects genetic analysis sample size: modernP. cookiiLBIn=26 and CDFn=19; historicalP. cookii BC n=9 and HCn=10. Figure 1: Pacific migrations of tracked P. cookii . Movements of P. cookii breeding on LBI (red circle, North Island) and CDF (purple circle, South Island), New Zealand. Approximate post-breeding and pre-breeding migration routes of tracked LBI (red dashed lines) and CDF (purple dashed lines) birds begin and end with mean migration departure and arrival dates (white text). Red and purple tones, and associated contour lines, represent the 95, 75, 50 and 25% kernel estimates for LBI and CDF birds respectively. Pie charts show the geographic distribution of cytochrome c oxidase subunit 1 mtDNA haplotypes sequenced from modern P. cookii populations (charts attached to LBI and CDF colony locations) and historical P. cookii skins collected in the North (BC) and South Pacific (HC) Ocean in 1905 and 1913 respectively (charts attached to white circles showing approximate collection location). Pie chart size reflects genetic analysis sample size: modern P. cookii LBI n =26 and CDF n =19; historical P. cookii BC n =9 and HC n =10. Full size image During initial eastward migration to South America, the routes taken by P. cookii from LBI and CDF overlapped, followed a similar direction to those of post-breeding sooty shearwaters ( Puffinus griseus ) [11] and Westland petrels ( Procellaria westlandica ) [30] , but not Australasian gannets ( Morus serrator ), departing from New Zealand nesting colonies [31] . Subsequently, LBI birds moved northwest across the equator and eventually returned on south-westerly trajectories to New Zealand along routes that were directionally similar to sooty shearwaters [11] , flesh-footed shearwaters ( Puffinus carneipes ) [32] and bar-tailed godwits ( Limosa lapponica baueri ) departing from on, or off, North America [33] . These observations highlight the existence of an important cross-taxa avian migration corridor within the Pacific Ocean between approximately 170°E and 160°W. Isotopic and habitat segregation P. cookii moult during the non-breeding period [26] , [34] , and hence incorporate local isotopic dietary signals in their new plumage [35] . Stable isotope ratios of C (δ 13 C) and N (δ 15 N) in particular provide an indication of carbon source (benthic versus pelagic, inshore versus offshore, and information on water mass) and trophic level of prey, respectively [35] , and comparisons thus can indicate geographic and/or dietary segregation [36] , [37] . Supporting the prediction that geographic divergence would be consistent between the P. cookii populations at a contemporary timescale (ca. 2–3 years), there was no significant difference in the isotope signatures of P. cookii body feathers collected in 2006 and 2008 from LBI (2006 untracked n =20, 2008 tracked n =11) (δ 13 C: Z=0.83, P =0.41; δ 15 N: Z=1.70, P =0.10) or CDF (2006 untracked n =20, 2008 tracked n =9) (δ 13 C: Z=1.34, P =0.19; δ 15 N: Z=1.79, P =0.07) ( Fig. 2 ) suggesting that currently, within each breeding population, birds forage within similar oceanic regions and on prey of a similar trophic level in successive years. 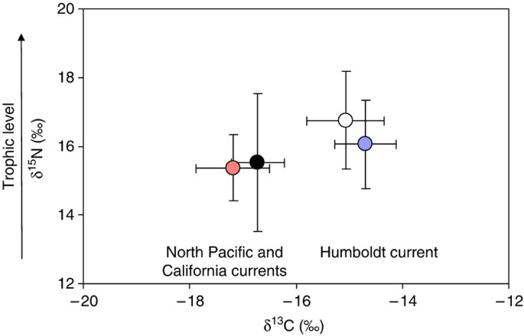Figure 2: Isotope ratios of contemporary and historicP. cookiifeathers. Feather isotope signatures ofP. cookii(±s.d.) from LBI (red circle, 2006 (untracked) and 2008 (tracked) combined,n=31) and CDF (purple circle, 2006 (untracked) and 2008 (tracked) combined,n=29) and from historical skins collected in the North Pacific (BC) (black circle, 1905,n=9) and South Pacific Ocean (HC) (clear circle, 1913,n=10). Figure 2: Isotope ratios of contemporary and historic P. cookii feathers. Feather isotope signatures of P. cookii (±s.d.) from LBI (red circle, 2006 (untracked) and 2008 (tracked) combined, n =31) and CDF (purple circle, 2006 (untracked) and 2008 (tracked) combined, n =29) and from historical skins collected in the North Pacific (BC) (black circle, 1905, n =9) and South Pacific Ocean (HC) (clear circle, 1913, n =10). Full size image In support of the prediction of a match between the stable isotope signatures of historical and contemporary samples sharing the same non-breeding provenance, variation in the δ 13 C signatures of feathers from modern (LBI: 2006 and 2008 combined; CDF: 2006 and 2008 combined) and historical specimens collected within the core non-breeding habitats of birds tracked from LBI and CDF, respectively (samples collected in 1905 at 22.42°N, 112.67°W, North Pacific Ocean, in the California Current region off Baja California, hereafter called BC, and in 1913 at ca. 11°S, 79°W, South Pacific Ocean, in the Humboldt Current, hereafter called HC; Supplementary Tables S1 and S2 ) suggest that birds have used population-specific oceanic regions, with similar carbon signatures, at historical time scales ( Fig. 1 ) (F=81.32, df=2, P <0.001). The mean δ 13 C value of LBI P. cookii (−17.18±0.70 s.d.‰) was not significantly different from that of historical samples from BC (−16.72±0.51 s.d.‰) ( t =2.085, P =0.250), but was significantly lower than that of modern samples from CDF (−14.69±0.58‰) ( t =14.92, P <0.01), and historical samples from HC (−14.79±0.73‰) ( t =9.292, P <0.001) ( Fig. 2 ). The mean δ 13 C value of modern CDF samples was not significantly different from that of historical samples collected within the HC ( t =0.42, P =1.00) but was significantly higher than historical samples collected from BC ( t =8.94, P <0.001) ( Fig. 2 ). These results suggest consistent differences in carbon isotopic signals between the North Pacific Convergence and South Pacific HC systems, and support our initial prediction. The mean δ 15 N value of modern LBI P. cookii feathers (15.37±0.95‰) was not significantly different from modern CDF feathers (16.05±1.29‰) ( t =3.69, P =0.16) and the only difference in mean δ 15 N value between modern and historical feathers was observed in modern samples from LBI (15.37±0.95‰) and historical samples from HC (16.76±1.42‰) ( t =3.53, P <0.01) ( Fig. 2 ). The most likely explanation for these results is that modern P. cookii feed on prey at similar trophic levels, despite occupying different oceanic regions (as suggested by tracking and carbon isotope data). Accordingly, the environmental characteristics of core non-breeding habitats exploited by modern LBI and CDF P. cookii were significantly different, with LBI P. cookii foraging over deeper (4930±581 s.d. m versus 3330±314 s.d. m, Z=−3.97, P <0.0001), warmer (20.11±1.97 s.d. °C versus 17.29±1.59 s.d. °C, Z=3.12, P <0.01) and less productive waters (0.16±0.10 s.d. mg Chl a m −3 versus 0.73±0.18 s.d. mg Chl a m −3 , Z=−3.91, P <0.0001) than their CDF conspecifics ( Fig. 3 ). At the intrapopulation level, comparisons of environmental characteristics for presence and absence data indicated that LBI P. cookii occupied less productive waters (0.16±0.10 mg Chl a m −3 versus 0.28±0.17 mg Chl a m −3 , Z=−2.20, P =0.03) and CDF P. cookii more productive waters (0.73±0.18 mg Chl a m −3 versus 0.47±0.12 mg Chl a m −3 , Z=2.79, P <0.01) than those available within their respective non-breeding core habitats ( Fig. 3 ). 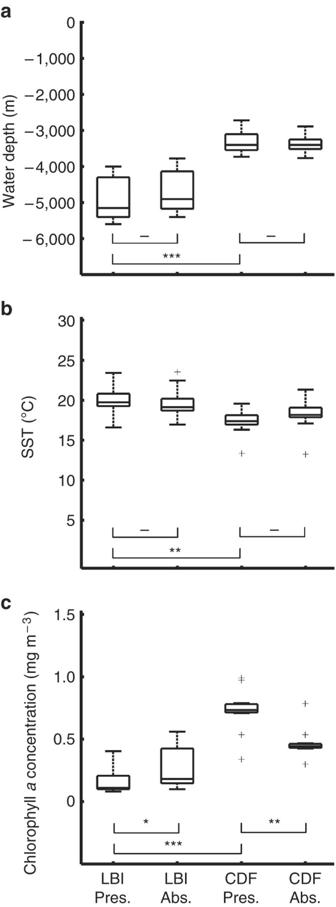Figure 3: Characteristics of selected oceanic habitats. Box plots of median values for remotely sensed environmental data (a. water depth,b. sea surface temperature,c. chlorophyllaconcentration) from logger locations ofP. cookiitracked from LBI (LBI,n=11) and CDF (CDF,n=11) during occupancy of core non-breeding habitats (LBI Pres. and CDF Pres., 20% UD) and in randomly selected proximate locations (LBI Abs. and CDF Abs.) seeMethods. Asterisks represent significance of difference for group comparisons: *P=0.05, **P=0.01, ***P=0.001, −=not significant. Box plots illustrate 25th, 50th (median), and 75th percentiles, error bars represent minimum and maximum values falling within 1.5 Inter Quartile Range, and crosses plot the outliers. Abs., absence; Pres., presence; SST, sea surface temperature. Figure 3: Characteristics of selected oceanic habitats. Box plots of median values for remotely sensed environmental data ( a . water depth, b . sea surface temperature, c . chlorophyll a concentration) from logger locations of P. cookii tracked from LBI (LBI, n =11) and CDF (CDF, n =11) during occupancy of core non-breeding habitats (LBI Pres. and CDF Pres., 20% UD) and in randomly selected proximate locations (LBI Abs. and CDF Abs.) see Methods . Asterisks represent significance of difference for group comparisons: * P =0.05, ** P =0.01, *** P =0.001, −=not significant. Box plots illustrate 25th, 50th (median), and 75th percentiles, error bars represent minimum and maximum values falling within 1.5 Inter Quartile Range, and crosses plot the outliers. Abs., absence; Pres., presence; SST, sea surface temperature. Full size image Genetic divergence Consistent with prediction that genetic analysis would confirm divergence in transequatorial migration of the P. cookii populations over historical timescales, all nine historical BC P. cookii skins had mitochondrial cytochrome c oxidase subunit 1 haplotypes that were identical to those of the modern LBI population [38] ( Fig. 1 ). Seven of ten historical HC P. cookii skins shared the same haplotype as that of modern CDF P. cookii [38] and each of the three remaining skins had a novel haplotype ( Fig. 1 ). We previously identified a single nucleotide polymorphism (at site 156) that differentiates modern LBI and CDF P. cookii [38] . All haplotypes sequenced from historical HC P. cookii skins in this study share the same diagnostic single nucleotide polymorphism as modern CDF birds, including the three novel haplotypes ( Fig. 1 , Supplementary Fig. S2 , Supplementary Tables S1, S2 and S3 ). These results support the previous predictions of contemporary and historical transequatorial separation of the extant P. cookii populations, revealed by our tracking and isotopic analyses, and suggests that these two populations have been genetically structured for a minimum of 100 years. Intrinsic factors that are argued to be restricting gene flow between seabird populations include natal philopatry [19] , divergent breeding timetables [39] , [40] and differences in breeding and non-breeding distributions [8] , [12] , [17] , though how these interact is poorly understood. Our combined results suggest that the use of population-specific non-breeding habitats has an interactive role in the restriction of gene flow, as both a pre-mating and a post-mating barrier. With regards to the former, migration routes of differing lengths or directions are widely recognized pre-mating barriers in migrant terrestrial bird species [5] , [41] , [42] . In P. cookii , differences in the duration of migratory movement or non-breeding distribution seem to underlie the pronounced breeding asynchrony between the populations. Moreover, regional differences in the timing of peak primary productivity, or the onset of gonad development based upon differences in day length and temperature shifts [43] , could amplify asynchronies in breeding timetables beyond those mediated by differences in route or non-breeding residency times alone. Thus, it is not spatial segregation during the non-breeding season per se. that represents a pre-mating barrier to gene flow. Rather, it is the interaction between differing non-breeding distributions and divergent breeding timetables, combined with high natal philopatry, that restricts gene flow. With regards to natal philopatry, adult Cook's petrel desert their chicks up to two weeks prior to fledging and, as seen in many migratory seabirds [5] , [41] , chicks presumably follow an inherited migratory direction and timing [5] , [42] . Studies of migrant terrestrial bird species indicate that the inheritance of suboptimal migration routes during secondary contact represents a post-mating barrier to gene flow [10] , [40] . Although secondary contact is presumably rare in P. cookii , the inheritance of an alternative or intermediate migratory strategy would place individuals at a selective disadvantage, if it led to the occupancy of suboptimal non-breeding grounds or breeding timetables that were out of synchrony with the rest of the population [10] , [40] . Habitat specialization during both the breeding and non-breeding season is also likely to promote divergence among the two extant P. cookii populations via local adaptation. For example, when breeding, P. cookii exhibit divergent, although overlapping, distributions and diets in response to regional differences in oceanography [25] . Moreover, the populations differ in body mass [22] with smaller LBI birds foraging in warmer low-latitude waters compared with larger CDF conspecifics [25] . That individuals from these two populations also occupy oceanic waters with similarly divergent characteristics during the non-breeding period (that is, LBI birds occupy warmer, less productive waters than CDF birds; Fig. 1 ) suggests population-specific adaptation to differing marine habitats, possibly linked to body size. Indeed, differences in seabird-habitat-use related to body size have been observed in other studies, particularly in species with pronounced sexual size dimorphism [44] , [45] , [46] . It remains uncertain whether body size differences between populations of P. cookii are a cause or consequence of divergent habitat use. Regardless, our data support and extend local adaptation hypotheses by suggesting that conspecific seabird populations can become tied to particular marine habitats during the breeding [18] , [39] , [47] and non-breeding periods, presenting ecologically driven opportunities for population divergence. Overall, this study demonstrates the use of integrative techniques to track inter-seasonal space use, behaviour, foraging ecology and to demonstrate clear spatial segregation of non-breeding distribution between two populations of seabird. This segregation is paralleled by divergent foraging ecologies and influences breeding phenology; it thus seems to represent an intrinsic barrier to gene flow, and has led to local adaptation in a highly mobile seabird. Tracking and environmental data P. cookii breeding on LBI and CDF were equipped with light-based loggers (British Antarctic Survey, Mk14) in November–December 2007 (LBI, 36° 11'S, 175° 04'E, n =13; CDF, 46° 11'S, 167° 38'E, n =14) during early incubation. Loggers were deployed on birds of known breeding history using established attachment techniques [25] with the total package weighing <1% of body mass. The sex of all birds were previously determined using molecular methods [25] , [48] . The following breeding season, 24 (89%) birds (LBI n =12 and CDF n =12) returned to breed and were recaptured in January–March 2009 at their same breeding burrows, and loggers were removed. Two loggers (LBI n =1 and CDF n =1) failed to download resulting in 11 datasets from each population for processing and analyses. Light data from the loggers were processed using Multitrace software (Jensen Software Systems) and locations (2 d −1 ) were estimated with an expected mean accuracy±s.d. of 186±114 km [49] . Sunrise and sunset times were identified based on light-curve thresholds, with latitude calculated from day/night length and longitude calculated from the time of local midday/midnight relative to Greenwich Mean Time. As a result of day-length uniformity around the equinoxes, clearly erroneous locations occurring 3–4 weeks either side of the equinox were excluded. Furthermore, points that involved movements of >1600 km in one day [50] , those with interruptions to light curves around sunset and sunrise, or that were clearly outside of the known or possible range for P. cookii , were removed from the data set. Totals of 7,886 and 9,082 locations were obtained for LBI and CDF P. cookii respectively, of which 9.7% and 10.6% were excluded after filtering. Filtered locations were then used to estimate year-round utilization distribution (UD) kernels for each population following methods detailed in ref. 51 . In brief, 2-D Gaussian kernel densities were estimated using custom routines created in MatLab [51] (The Mathworks). Kernels were calculated using a Lambert Cylindrical Equal Area projection on an 80 km grid with grid cells normalized for bird effort by dividing each cell by the number of birds contributing the locations within a cell. The kernel smoothing parameter (h) was estimated using an adaptive method [52] to estimate an optimal local value, following ref. 53 . Based on published methods [25] , a 1,000 km buffer was used around each colony to define breeding habitat, and the 80% contour of UD kernels, calculated individually, were used to define the core non-breeding distributions for each bird [50] . Dates of the first and last locations to enter and exit the core non-breeding habitats were used to define migration timing for each individual. Individuals' migration distances were calculated by summing the point-to-point distances travelled during post-breeding and pre-breeding movements between these core areas. Satellite-derived remotely sensed environmental data were used to contrast the core habitats of P. cookii from LBI and CDF during the non-breeding period (presence dataset) as well as those available, but not used, within each population-specific region (absence dataset). For the presence dataset, environmental data were extracted for logger locations falling within the 20% UD for each tracked bird using a 1° longitude by 2° latitude grid centred (the approximate error of geolocation estimates) on the date and coordinates of the location [51] . For the absence dataset, environmental data were extracted from ten randomly selected locations, derived within a 1,000 km radius buffer of each logger location and centred on the corresponding logger location date. Environmental data extracted for the random locations were averaged to give a mean absence estimate to contrast presence values. Remotely sensed environmental data were obtained from NOAA's Environmental Research Division ( http://swfsc.noaa.gov/erd.aspx ) including 5-day composites of chlorophyll a (Chl a ) concentration (mg Chl m −3 ) at a spatial resolution of 0.1° resolution [54] and 8-day composites sea surface temperature in °C with a spatial resolution of 0.1° (ref. 55 ). Bathymetric data were obtained from the ETOPO2 dataset [56] . Stable isotopes To contrast population-specific dietary signals during the non-breeding period, we conducted stable isotope analyses of C (δ 13 C) and N (δ 15 N) ratios in body feathers collected from modern LBI and CDF P. cookii and museum specimens held at the Californian Academy of Sciences ( n =9) and American Museum of Natural History ( n =10). Single body feathers were collected from breeding P. cookii in 2006 and from tracked birds upon their recapture in 2009, with no resampling of birds between years. Modern and historical feathers were cleaned with 70% ethanol, then washed in distilled water to remove contaminants, dried in at 50°C and cut into fine fragments using scissors. Stable isotope analyses of δ 15 N and δ 13 C, using a subsample (approximately 0.7 mg) of each homogenized feather, were carried out on a DeltaPlus (Thermo-Finnigan) continuous flow isotope ratio mass spectrometer using protocols outlined by ref. 25 . Measurement precision of the isotope analysis was 0.29‰ for δ 15 N and 0.24‰ for δ 13 C. To account for the Seuss effect, the temporal biasing of the atmospheric CO 2 pool to more negative δ 13 C values as a result of the burning of fossil CO 2 , δ 13 C data from historical feathers where normalized by subtracting a year-specific factor δ 13 C=−1+1.1 (2009-year (1905 or 1913))*0.027 following ref. 57 Genetic analyses Toe pad skin samples were collected from the same historical Cook's petrel specimens from which feathers were sampled for stable isotope analyses ( Supplementary Tables S1 and S2 ). DNA extraction and polymerase chain reaction set up was performed in a physically isolated, dedicated ancient DNA laboratory. Contamination was monitored using extraction and PCR negative controls and genomic DNA was isolated as per ref. 58 . A 375 base pair (bp) region of the mitochondrial cytochrome c oxidase subunit 1 gene was amplified using two sets of primers that amplified two overlapping fragments: AWCF1 and AWCintR2 (ref. 58 ); LCRintF2 5′-TCATAATTGGGGGATTTGGA-3′ (designed using Primer3 software [59] ) and AWCintR3 (ref. 58 ). This region corresponds to the first 375 bp of the 677 bp fragment sequenced by ref. 38 . PCR products were purified using a QIAquick PCR Purification kit (Qiagen) then sequenced bidirectionally from independent PCRs [58] . Sequences were concatenated and aligned using Sequencher version 4.8 (Gene Codes), deposited in NCBI GenBank (accession numbers HQ263645 to HQ263663 ) and compared with those in ref. 38 . Statistical analyses Habitat data extractions, processing and analyses were conducted using Matlab (The Mathworks). Non-parametric Mann-Whitney U tests were used to test for differences between presence and absence habitat data for the extracted environmental parameters at an intra-population level, and for the presence data at an interpopulation level. Mean environmental parameter values for individual birds were used as the sampling unit. Mann-Whitney U tests were initially used to compare stable isotope values between years (2006 and 2009) for LBI and CDF. Isotope data (δ 15 N and δ 13 C) were subsequently pooled for each population and permutation-based non-parametric ANOVA, with pair-wise comparisons using the Bonferroni correction method, conducted to compare isotope values between individuals from the breeding populations (LBI and CDF) and museum skin specimens (CAS 1905 and AMNH 1913) using the programme PERMANOVA. Sex was initially included as a factor in all analyses, but excluded as a result of nonsignificant differences. How to cite this article: Rayner, M.J. et al . Contemporary and historical separation of transequatorial migration between genetically distinct seabird populations. Nat. Commun. 2:332 doi: 10.1038/ncomms1330 (2011).